Probing biomechanical properties with a centrifugal force quartz crystal microbalance Application of force on biomolecules has been instrumental in understanding biofunctional behaviour from single molecules to complex collections of cells. Current approaches, for example, those based on atomic force microscopy or magnetic or optical tweezers, are powerful but limited in their applicability as integrated biosensors. Here we describe a new force-based biosensing technique based on the quartz crystal microbalance. By applying centrifugal forces to a sample, we show it is possible to repeatedly and non-destructively interrogate its mechanical properties in situ and in real time. We employ this platform for the studies of micron-sized particles, viscoelastic monolayers of DNA and particles tethered to the quartz crystal microbalance surface by DNA. Our results indicate that, for certain types of samples on quartz crystal balances, application of centrifugal force both enhances sensitivity and reveals additional mechanical and viscoelastic properties. There are few experimental techniques that allow the study of force on biological molecules. Among them, optical or magnetic tweezers and atomic force microscopes (AFMs) have provided much insight into the mechanics of DNA, RNA and chromatin [1] , [2] , [3] , [4] , friction and wear in proteins [5] , [6] and stepwise motion of motor proteins [7] , all of which are important for understanding disease. However, powerful, these methods have difficulty operating as integrated devices to probe the mechanical properties of heterogeneous samples in a wide range of applications in situ and in real time; tweezer and AFM experiments rely on highly trained experimentalists, are not widely applicable as analytical tools and are often constrained to the analysis of well-prepared, homogeneous samples. Among direct mechanical transduction methods amenable for biosensing, the quartz crystal microbalance (QCM) has seen great utility as a simple, cost effective and highly versatile mechanical biosensing platform. Since its introduction by Sauerbrey [8] in 1959 as a thin-film mass sensor in the gas phase, the understanding and real-world applicability of these devices have been repeatedly enhanced to study phenomena such as viscoelastic films in the liquid phase [9] , contact mechanics [10] and complex samples of biopolymers and biomacromolecules [11] . Naturally, these benefits do not come without disadvantages. The underlying mechanical properties of the sample that occur on loading of the biomaterial are often not revealed by the stepwise changes in the QCM sensorgram, an issue complicated by the choice of theoretical model. Here we introduce a novel QCM-based biosensing technique that enables monitoring the mechanical response of a sample to the continuous application of a variable centrifugal force. This centrifugal force quartz crystal microbalance (CF-QCM) concept enables direct introduction of pico- to nanoscale forces in the liquid phase for analysing a sample’s mechanical properties. We show that the response of a sample under centrifugal load is revealing of its viscoelastic, mechanical and conformal properties. Experiment The experimental set-up under consideration is shown schematically in Fig. 1a . It consists of a QCM integrated into the arm of a commercial swinging bucket centrifuge. The QCM is connected in proximity to a remote driver, which is tethered via a slip-ring connector to external data acquisition electronics. The crystal itself is mounted in a holder radially by its edges such that the centrifugal force F c is always normal to the surface of the crystal. On the sensing side of the crystal is a 125-μl volume PDMS/glass cell containing the sample. The non-sensing side of the crystal remains in air. When in operation, the crystal and cell are mounted either in the loading configuration, where the centrifugal force is in to the sensing side or, by mounting it upside down, in the unloading configuration, where the force is away from the sensing side. 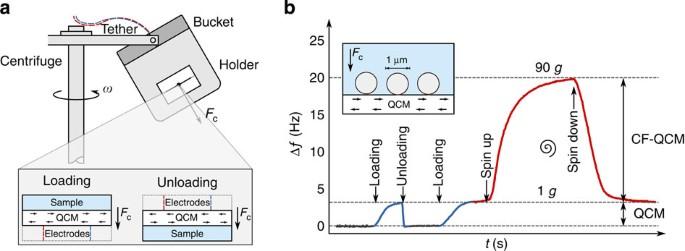Figure 1: Overview of the CF-QCM. (a) Experimental set-up. A QCM and its driver are integrated into one arm of a standard swinging bucket centrifuge. Data acquisition is done electrically through a tether and a centrally mounted slip ring. When spinning, centrifugal force is applied to a sample under assay. Here, whereac=ω2Randagare centripetal and gravitational accelerations, respectively. (b) Example CF-QCM experiment with 1 μm particles in water,NL=1.58 × 1011particle m−2, in the ‘loading’ configuration (inset). The horizontal arrows indicate the motion of the QCM transverse shear mode. The spin up to 90gin loading configuration enhances the QCM frequency shift signal and allows extraction of mechanical properties of the sample, as well as particle size. See text for details. Figure 1: Overview of the CF-QCM. ( a ) Experimental set-up. A QCM and its driver are integrated into one arm of a standard swinging bucket centrifuge. Data acquisition is done electrically through a tether and a centrally mounted slip ring. When spinning, centrifugal force is applied to a sample under assay. Here , where a c = ω 2 R and a g are centripetal and gravitational accelerations, respectively. ( b ) Example CF-QCM experiment with 1 μm particles in water, N L =1.58 × 10 11 particle m −2 , in the ‘loading’ configuration (inset). The horizontal arrows indicate the motion of the QCM transverse shear mode. The spin up to 90 g in loading configuration enhances the QCM frequency shift signal and allows extraction of mechanical properties of the sample, as well as particle size. See text for details. Full size image An example CF-QCM response for free particles is depicted to the left in Fig. 1b . Here, free 1 μm streptavidin-coated polystyrene particles in water are introduced into the sample cell. When the cell is rotated to the loading configuration under the influence of gravity alone, the particles fall towards the sensing surface and a positive shift in the QCM’s frequency signal is observed. When the cell is then rotated 180° to the unloading configuration, the particles fall off and the frequency response returns to its original state. Again the cell is rotated 180° to the loading configuration and the positive frequency shift is observed. As the centrifuge spins up towards 90 g , the particles are ‘pressed’ towards the QCM surface and a fourfold increase in the frequency shift is observed. The centrifuge then spins down and the baseline frequency shift under gravity alone is recovered. Traditional QCM experiments assume that the inertial properties and rigidity of the sample coupling are taken as a fixed parameter (or statistical distribution) under assay. With this approach, however, one is only able to obtain discrete values in an otherwise continuous parameter space. Hybrid-QCM experiments involving nanoindenters [12] or AFM probe tips [13] have shown intriguing behaviour when force is applied to a sample in a QCM measurement. There have also been reports that accelerations as small as 1 g have a measurable effect on a QCM response for viscoelastic monolayers such as DNA [14] , and even for pure Newtonian liquids [15] . All of these responses have been found to be significant compared with the baseline acceleration sensitivity of the QCM itself [16] . With the integration of a centrifuge to a standard QCM, one can observe these effects under enhanced g-forces and make end point measurements (measurements taken after the addition of a sample) in the sample’s parameter space continuously and repeatedly. To demonstrate this, we have examined six different samples in the CF-QCM under variable accelerations from ~1–90 g . These samples were chosen to be examples of the breadth of load situations accessible with our technique. They are (a) air, (b) deionized water, (c) free particles in water, (d) paramagnetic particles attached to the sensor via short oligonucleotides, (e) 48-kbp lambda phage DNAs attached to the gold electrode and (f) polystyrene particles tethered to the sensor via 48-kbp lambda phage DNAs. The employed QCM driver circuit outputs Butterworth van Dyke (BvD) equivalent relative frequency Δ f (in hertz) and motional resistance R (in ohms). R is approximately related to the bandwidth Γ (half width at half maximum of the frequency response) by Γ= R /(4π L ), where L =40 mH is the motional inductance of the BvD equivalent circuit [17] . For this relationship we assume the small load approximation Δ f / f F ≪ 1, where f F is the fundamental frequency [18] . It is therefore relevant to note our assumption that Δ R is an approximate, and indirect, measure of the bandwidth ΔΓ (in hertz). In addition ΔΓ is an equivalent representation of the ‘dissipation’, D , used in QCM-D devices by D =2ΔΓ/ f F (See Supplementary Note 1 ). The instrument’s response was first tested in air, shown in Fig. 2a . The base acceleration sensitivity (change in frequency versus change in g-force) of AT cut quartz normal to the plane of the crystal has a reported value [19] of Δ f /Δ g =2.188(6) × 10 −2 Hz g −1 . Our instrument shows similar behaviour: Δ f /Δ g =2.682(23) × 10 −2 Hz g −1 in the loading configuration. The signs of Δ f /Δ g are found to be opposite in the loading and unloading configurations. We have not found a reference for the bandwidth or motional resistance dependence of a QCM under acceleration, but we find the value to be ΔΓ/Δ g =9.203(171) × 10 −4 Hz g −1 . 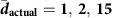Table 2 Results of the particle sizing method applied to particles with diametersand 25μm. No description available Figure 2: Load situations. Change in frequency Δ f and bandwidth ΔΓ (in hertz, inferred from motional resistance) of the CF-QCM under different load situations as the centripetal acceleration is directed in to (loading, represented by circles with the top half colored) and out of ( unloading , represented by circles with the bottom half colored) the plane of the crystal. The situations are ( a ) unloaded crystal in air, ( b ) deionized water, ( c ) free 1-μm diameter streptavidin-coated polystyrene particles, N L =1.58 × 10 11 particle m −2 , ( d ) 2 μm diameter streptavidin-coated paramagnetic particles, N L =1.65 × 10 10 particle m −2 , attached with 25mer oligonucleotides, ( e ) lambda DNA only attached to the gold electrode and ( f ) 25 μm diameter streptavidin-coated polystyrene particles, N L =3.25 × 10 7 particle m −2 , tethered to the sensor surface with 48-kbp lambda DNAs. Error bars are derived from uncertainties (standard deviation) in the centrifuge both spinning up and spinning down in a single experimental run. Full size image Next, deionized water was used as a control sample for measurement in the liquid phase, as shown in Fig. 2b . The initial shift in frequency and bandwidth is in agreement with what is obtained from the Kanazawa-Gordon relations [9] for water ( ρ =1 g cm −3 and η =1 mPas): Δ f =−714 Hz and R =359 Ω, which are close to the measured values of Δ f = −716 Hz and R =357 Ω. The response under centrifugal load was found to be linear and smaller than that of air: Δ f /Δ g =1.357(24) × 10 −2 Hz g −1 and ΔΓ/Δ g =2.865(73) × 10 −3 Hz g −1 . We observe that these acceleration-dependent forces in the liquid phase are not necessarily commensurate with those in the gas phase, but, as the effects are small compared with experiments with actual loads, we treat them as baselines to be subtracted. Utilizing the flexibility that the instrument provides in modifying the coupling between the load and the sensor surface, we have applied the technique to the study of discrete micron-sized particles. As first referenced in Fig. 1b , the frequency and bandwidth shifts of free particles in the liquid phase as a function of g-force is shown in Fig. 2c . Here, streptavidin-coated polystyrene particles, mean diameter , are placed in the sample volume with a surface density of N L =1.58 × 10 11 particle m −2 . and the signal is observed in both the loading and unloading configurations. The particles did not exhibit adhesion to either the unmodified gold electrode or the glass/PDMS cell surrounding it; in the unloading configuration, the particles quickly drifted away from the sensing area and a signal identical to water was observed. In the loading configuration, a large positive shift in Δ f and ΔΓ was observed, consistent with previously observed responses for weakly coupled particles in this size range [10] . The initial shift under 1 g was found to be Δ f =2.2 Hz and ΔΓ=7.5 Hz. At the maximum acceleration of 90 g the signal increases to Δ f =16.5 Hz and ΔΓ=37 Hz. This also represents a sensitivity enhancement in the minimum resolvable surface density of the particles. The scaling of Δ f and ΔΓ with increasing centrifugal load is nonlinear in the applied load, implying non-Hertzian behaviour [12] . The same experiment was also carried out with 2, 6, 15 and 25 μm polystyrene particles. The loading curves all followed the same trend, but the relative shifts in Δ f and ΔΓ differed based on particle size. The results from these loads are summarized in Table 1 . Table 1 Normalized frequency and bandwidth shifts (in Hz m 2 ) at 1 and 90 g for various particle sizes in water. Full size table In contrast to the situation of free particles, we have also studied the behaviour of the CF-QCM in a regime where particles are rigidly coupled to the sensor by attaching 2 μm (mean diameter ) streptavidin-coated paramagnetic particles modified with biotinylated 25mer oligos to complimentary strands conjugated to the QCM gold surface via thiol bonds (see Materials). This is shown in Fig. 2d . Note that, Δ f and ΔΓ are both negative and decrease with centrifugal force in the loading orientation. When spinning with the oligo-attached particles, we suspect we are not sensing the presence of the particle directly but rather the conformational state of the oligonucleotide layer. Such an acceleration effect has been observed before [14] , [15] , but only within the 2 g orientation difference of gravity. When the oligo layer is under centrifugal load, it compresses, causing the density–viscosity product to increase. This behaviour is consistent with the behaviour of DNA observed on QCMs under the influence of gravity alone [14] . Moving from particles to viscoelastic monolayers, in Fig. 2e , 48-kbp lambda phage DNA in STE buffer was attached to the gold sensor electrode via a complimentary thiolated oligo. Previous studies have shown that, through the use of dissipation monitoring, QCMs are sensitive to not only the adsorbed mass and viscosity, but the physical conformal state (‘shape’) of DNAs hybridized to the sensor surface [20] . In the experiment, even though the force on the lambda DNAs is on the order of femtonewtons, we observe a strong linear decrease (ΔΓ=−2.9120(95) Hz g −1 ) in the bandwidth as function of g-force, indicating an increase in viscoelastic loss. However, under larger g-forces the sign of Δ f reverses. The origin of this effect is not understood, but could indicate a nonlinear viscoelastic compliance under load. The unloading configuration sees a smaller negative response in ΔΓ with little effect on Δ f . At this point we make an observation about the influence of salt buffer, which was used in experiments involving DNA. There are several studies [21] , [22] regarding the effects of various electrolytic buffer solutions and their concentrations on QCM measurements, including reports of an immersion angle (and therefore gravity) dependence [23] . These reports suggest this effect may be related to the behaviour of the interfacial layer and ion transport in monovalent electrolytic solutions in accelerating frames [24] , [25] . We have observed a significant contribution in the unloading configuration for STE buffer alone (Δ f = −0.3260(29) Hz g −1 , and ΔΓ nonlinear), which was subsequently ‘screened’ [26] by the presence of both oligos and lambda DNAs, making the effect negligible in the current set of experiments. Further investigation is required to explain this precisely. With the sensitivity to both particles and monolayers, the instrument raises a possibility for using beads tethered by lambda DNA as a transduction mechanism to investigate its kinetics. One such example is shown in Fig. 2f . Streptavidin-coated polystyrene particles with a mean diameter of 24.8 μm were tethered to the CF-QCM by means of a 48-kbp lambda phage DNA. Experiments were carried out in STE buffer whose density reduced the maximum force the bead could exert to about 40 pN, which, according to the worm-like chain model [4] , should almost fully extend the lambda DNA to a length of 16 μm. Although the instrument has not yet been developed enough to make accurate quantitative measurements in this load situation, the behaviour of the data is a clear indication of its potential. As the tethered bead extends the DNA under centrifugal force, Δ f increases and ΔΓ decreases. In the case where the DNAs are trapped and pushed between the bead and the surface, both Δ f and ΔΓ increase. We have confirmed the signs of the shifts in this scenario with 10 and 6 μm paramagnetic particles, using a magnet to either pull or push the particles towards or away from the sensor surface. This behaviour is distinct from either the case of lambda DNA or the free particles alone. At F c =40 pN, the frequency shift indicates an effective decrease in the density–viscosity product of 10% or about 1.5 pg. For the surface densities involved ( N L =3.25 × 10 7 particle m −2 ), the equivalent interfacial mass lost for a fully extended lambda DNA predicted by the worm-like chain model is in the picogram range and cannot account for the >10 6 signal difference shown here. If indeed the response is due to lambda DNA extension, future experiments involving high frequency, large centrifugal force CF-QCMs could easily detect the kinetics of a single tether. Theory and modelling To elucidate QCM behaviour for samples with discrete particles, we have performed 2D finite element simulations based on steady-state solutions to the incompressible Navier-Stokes equations. This model and its implementation are described in Supplementary Note 2 . The simulation is set up as depicted in Fig. 3a–c . Particles are represented as spheres (or rather cylinders, in 2D, see Supplementary Fig. 1 ), which are moved towards a tangentially oscillating boundary at the bottom of the computational domain, representing the QCM surface. Periodic conditions are imposed on the left and right boundaries such that the ratio of the domain width to the particle size determines the surface coverage and thus N L . As the particle intersects the oscillating boundary it is truncated; we identify this truncation with a finite contact radius r c in terms of contact mechanics. 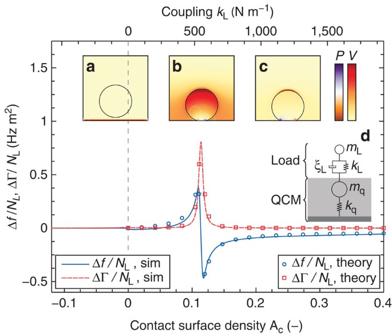Figure 3: Simulation of the CF-QCM behavior. Finite element simulation for a 10-μm polystyrene sphere (cylinder in 2D) as a function of contact surface densityAc. Negative values ofAcindicate positive separation from the surface. Discussion in the text. (a–c) Density plot of the pressurePand velocityUdistributions. Units are normalized. Note that in all situations with finite contact radius, stress is annularly distributed around the edge of the contact as per the Mindlin model48. (main plot): Shifts in Δfand ΔΓ. (d) Mechanical model based on coupled oscillators. Points on the plot are a best fit of the mechanical model to the simulation. Figure 3: Simulation of the CF-QCM behavior. Finite element simulation for a 10-μm polystyrene sphere (cylinder in 2D) as a function of contact surface density A c . Negative values of A c indicate positive separation from the surface. Discussion in the text. ( a – c ) Density plot of the pressure P and velocity U distributions. Units are normalized. Note that in all situations with finite contact radius, stress is annularly distributed around the edge of the contact as per the Mindlin model [48] . (main plot): Shifts in Δ f and ΔΓ. ( d ) Mechanical model based on coupled oscillators. Points on the plot are a best fit of the mechanical model to the simulation. Full size image A plot of the simulated response in frequency and bandwidth for a 10-μm particle is depicted in Fig. 3 . The spheres were modelled as polystyrene with density ρ =1.06 g cm −3 , shear modulus | G L |=1.3 GPa and loss tangent tan δ =0.001. The spheres are in water with density 1.0 g cm −3 and viscosity 1.0 mPa s. The shifts in Δ f and ΔΓ are plotted as a function of a dimensionless contact surface density A c , defined as the contact area of the sample per unit area on the oscillating boundary. The behaviour of the simulation closely matches experimental observations. As the sphere approaches and makes (weak) contact with the oscillating boundary, a positive shift in both frequency and bandwidth is observed. As the contact radius increases, the sphere becomes more strongly coupled to the boundary. The amount of energy dissipated into the particle increases until ΔΓ reaches a maximum and Δ f experiences a zero crossing. The limiting case sees a rigid attachment and the common negative frequency shift proportional to mass adsorption takes hold. There are two aspects of the simulation that deserve additional consideration: (1) positive shifts in Δ f and ΔΓ begin before physical contact with the oscillating boundary and (2) for smaller particles ΔΓ>Δ f while for larger particles Δ f >ΔΓ. The experiment shows the same behaviour, as evidenced in Table 1 . We note, however, that the procedure of truncation and its interpretation as finite contact radius in the framework of contact mechanics utilized here on discrete objects are more accurate for larger particles (10 μm, as shown in Fig. 3 ) than smaller ones. We explain this in the following way. It is known in the context of DVLO theory [27] that a micron-sized polystyrene sphere in water near a similarly charged gold surface will experience a repulsive force due to electrostatic double-layer effects [28] , [29] . The balance between this and the gravitational force determines the height at which the particle will be at equilibrium above the surface. For the relevant material parameters [27] , [30] we find that, even at 90 g , the smaller 1 and 2 μm particles never make contact with the surface, but ‘hover’ at separations of ~0.3–0.15. At non-zero separations we posit that the sphere-surface coupling, being mediated by a viscous liquid, will be dominated by loss, hence ΔΓ>Δ f . In contrast, larger particles (~10 μm and above) with significant mass will overcome the double-layer forces and make contact with the QCM through a finite contact radius. In this case the coupling losses decrease and Δ f >ΔΓ. Without mention of the actual physics of the coupling, we observe that the finite element simulation, as well as the experimental data, follows a simple mechanical model based on coupled oscillators [31] , [32] . The arrangement of this mass-spring-dashpot mechanical model is shown in Fig. 3d . Here, the resonance of the quartz crystal is coupled to a sample load with mass m L though a parallel spring k L and dashpot ξ L (Voigt model [33] ). Note that k L is not an actual spring; it is simply a coupling strength between two oscillators. The same is true for ξ L . m L is an actual mass, though in this model it represents a Sauerbrey mass uncorrected for viscoelastic properties. Using the small load approximation, the response of the system as a function of its coupling k L can be expressed as [34] where Z q is the acoustic impedance of AT cut quartz, f F is the fundamental frequency of the resonator and N L is a surface density (number per unit area) for discrete loads. Equation (1) as a function of k L reproduces the response of the finite element simulation in Fig. 3 , which is a function of contact surface density A c (or in un-normalized terms the contact radius r c ). A best-fit comparison with the finite element simulation is shown as points in conjunction with the simulation in Fig. 3 . See Supplementary Note 3 . The mechanical model has two important limits as a function of the contact stiffness, k L , known as strong and weak coupling. These limits occur to the left and right of a zero crossing in Δ f at . where we have made the approximation that ξ L ≪ k L (ref. 34 ). Strong coupling is identified with mass loading (Sauerbrey [8] behaviour) and a negative frequency shift linearly proportional m L . This behaviour is the one that is most commonly associated with QCM measurements. Physically this situation is identified with a coupling rigid enough such that the particle takes part in the oscillation of the QCM. In the opposite limit is weak coupling, also called inertial loading [31] , and is identified by a positive frequency shift independent of the mass and linearly proportional to k L . Here, the coupling is sufficiently weak such that the particle remains at rest in the labratory frame. It is ‘clamped’ by its own inertia [35] . Experiments with nanoindentation probes operating on QCMs in the gas phase [12] , where micron-sized spherical tips are pressed against the sensor surface, have observed the same positive frequency shift as a function of applied force, which is identified with the lateral (sphere-plate) Hertzian spring constant. We conjecture that similar behaviour will be observed in the liquid phase: the centrifugal load will primarily act on k L . We now turn to discussion of how certain sample parameters can be extracted using this model. The response of the QCM for different load situations under centrifugal force exhibits a rich and complex set of behaviour. Interpretation of all signals will require experiments beyond the scope of this manuscript, but we comment on a few examples where our preliminary data can be predictive within the general model we have set forth. The coupled oscillator model (equation (1)), when analysed for samples of free particles ( Figs 1b and 2c , and Table 1 ), suggests an avenue to allow QCMs to determine the size of large micron-sized particles in the liquid phase. Thus far, this has only been possible with nanometre-sized particles, which lie within the QCM’s shear acoustic wave [36] . If one plots Δ f versus ΔΓ in equation (1) as a parametric function of k L , the points are found to lie on a circle with radius r L . In doing so, the physical mechanism modifying k L is removed from the problem. If we then fit a circle to the experimentally observed Δ f –ΔΓ data (plotted parametrically as a function of g-force), we can extrapolate the behaviour in the strong coupling regime by finding the point at which ΔΓ=0 and Δ f <0. Knowing Δ f , equation (3) can then be inverted to solve for either number density or particle size/mass. An example of this procedure is shown in Fig. 4 using the same data for 1 μm particles shown in Figs 1 and 2 . Inset is a table for the same predictions done for particles with known diameter . In all cases the surface density was known and the diameter was derived from the mass m L , found by inverting equation (3). The results are surprisingly accurate despite the exploratory nature of the instrument’s construction, which illustrates the robustness of this unique methodology that CF-QCM provides. It should also be mentioned that with knowledge of the way in which the g-force modifies k L , the frequency zero crossing at can be used to determine the mass m L without knowledge of the number density N L . Finally, we comment on the potential of the CF-QCM technique to be sensitive to different viscoelastic properties of discrete samples. While the mechanical properties seen in biomaterials span an enormous range [37] , we choose three general categories to highlight potentially interesting sensor responses. As per Fig. 5 these are as follows: cells [38] , agarose microparticles [39] , [40] and protein microcrystals [41] . Each is treated in the finite element simulation as a discrete sphere, with complex shear modulus , where is the storage modulus related to elasticity and is the loss modulus related to viscosity. G L is related to viscosity η L by η L = G L /( iω q ). The shifts in frequency Δ f and bandwidth ΔΓ are again plotted as a function of the dimensionless contact surface density A c . A fictitious negative A c is identified with a finite separation distance from the simulated QCM surface. In all cases, the coverage ratio was 50%, and furthermore we assume that centrifugal force will act to ‘push’ the sample into the QCM surface, increasing A c and thus the rigidity of its contact with the QCM. 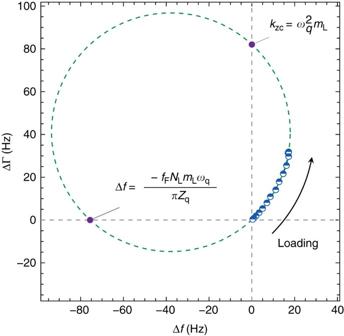Figure 4: Particle sizing. Method for sizing micron-sized particles using the CF-QCM. Δfversus ΔΓ is plotted parametrically as a function of g-force, and the data are fit to a circle. The point on the circle for which ΔΓ =0 and Δf<0 provides an estimate of mass adsorption, and thus particle size. Results for particles with diametersare shown inTable 2. Fit circle has a radius of 55.77 Hz and a center of (−37.83, 41.05) Hz. Figure 4: Particle sizing. Method for sizing micron-sized particles using the CF-QCM. Δ f versus ΔΓ is plotted parametrically as a function of g-force, and the data are fit to a circle. The point on the circle for which ΔΓ =0 and Δ f <0 provides an estimate of mass adsorption, and thus particle size. Results for particles with diameters are shown in Table 2 . Fit circle has a radius of 55.77 Hz and a center of (−37.83, 41.05) Hz. 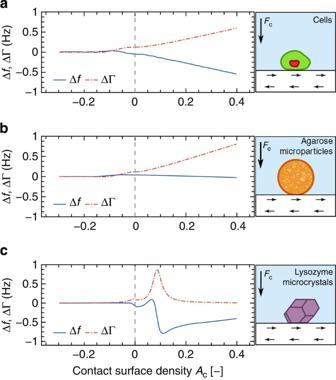Figure 5: Simulated response for different materials. Finite element simulation of normalized Δfand ΔΓ for three categories of samples as a function of contact surface density,Ac. Negative values indicate the sample has not made contact with the sensor surface. The samples are (a) cells,GL=(10+50i) kPa, (b) agarose microparticles,GL=(78+78i) kPa and (c) lysozyme microcrystals,GL=(0.659+0.235i )GPa. Full size image Figure 5: Simulated response for different materials. Finite element simulation of normalized Δ f and ΔΓ for three categories of samples as a function of contact surface density, A c . Negative values indicate the sample has not made contact with the sensor surface. The samples are ( a ) cells, G L =(10+50i) kPa, ( b ) agarose microparticles, G L =(78+78i) kPa and ( c ) lysozyme microcrystals, G L =(0.659+0.235i )GPa. Full size image As can be seen, the simulated response of the CF-QCM is markedly different in each case. Cells, shown in Fig. 5a , are assigned a shear modulus of G L =(10+50i) kPa and density ρ L equal to the surrounding liquid medium. The high loss modulus and low storage modulus predict that the cell will exhibit shifts characteristic of a viscous fluid. Similarly, the simulation shows Δ f and ΔΓ decrease and increase linearly proportional to the contact parameter, beginning before physical contact occurs. The proportionality is a simple function of the shear modulus and density in the semi-infinite approximation [9] , [42] Cells in and of themselves span a large range of viscoelastic properties, which have been demonstrated to be predictive for diseases such as cancer [43] . If one knows the way with which A c is modulated by an applied force (for example, viscoelastic compliance), linear fitting to the CF-QCM response will recover G L or ρ L . Next, Fig. 5b shows the simulated response of agarose microparticles with a complex shear modulus of G L =(78+78i) kPa. Again the density was assumed to be the same as the surrounding medium. Similar to the viscous behaviour of cells, ΔΓ decreases linearly with A c . In this sample, however, an equally large elastic term, , precludes the equally linear decrease in Δ f seen for cells. Instead, Δ f increases slightly before contact and then decreases slightly. At the end of the spectrum are lysozyme microcrystals, shown in Fig. 5c . These microcrystals are ‘hard’, having been assigned a complex shear modulus of G L =(0.659+0.235i) GPa. The response of these is similar to what we experimentally observe with polystyrene microparticles ( G L =1.3 GPa). When the microcrystal enters the acoustic evanescent wave, there is an initial negative shift as the effective viscosity–density product increases. At small contact parameters there is a positive shift in Δ f and ΔΓ. Increasing the contact parameter, ΔΓ sees a maximum and Δ f a zero crossing. As the microcrystal becomes strongly coupled to the QCM, the familiar negative Δ f is recovered which, as in Fig. 4 , can be used to determine the particle size or mass. We have observed the QCM sensorgram under the influence of centrifugal force for samples such as DNA monolayers, free discrete polystyrene particles and particles tethered to the QCM electrode with lambda DNA. We present simulations and a theoretical framework to interpret the QCM signals in the context of the sample’s properties. The data presented thus far point to a potentially interesting avenue for the investigation of force on biomolecules using a quartz crystal microbalance. In addition to the data discussed, we have also observed other types of signals in some of our data sets within the overall trend shown here, which we suspect may be related to ionic transport [24] , [25] , the conformal state of DNA and nonlinear viscoelastic behaviour. Objects such as microparticles attached or tethered to a biopolymer on the QCM surface become inertial transducers through which one can extract mechanical and thermodynamic properties of the macromolecules. Furthermore, the technique is applicable to microscopic biological objects such as viruses, bacteria and cells where measurements of mechanical properties and their changes have been directly linked to disease [44] , [45] , [46] . The enhanced signal for most samples under centrifugal load points to an interesting avenue of increasing the sensitivity of a state of the art QCM biosensor. This is true even with the present state of our instrument, which is limited to low-g regimes when compared to other commercial centrifuges. With operation below 90 g , we have observed sensitivity increases corresponding to changes of 10% in the density–viscosity product for viscoelastic loads, and up to a factor of 10 increase in sensitivity for discrete particles. However, there is no technical reason why future incarnations could not spin much faster and considerably clarify the CF-QCM sensogram. There are also possibilities in using this platform in other related modalities such as the nanotribological effects of sliding friction [47] caused by orienting the crystal at an angle to the applied centrifugal force, propelling biomolecules across the surface. Setup The experimental set-up used a 25-mm diameter 5 MHz gold-coated crystal in combination with an SRS QCM200 PLL based driver circuit. On the sensing side of the crystal is a 125-μl PDMS/glass cell containing the specimen under investigation. The cell is made of a thin o-ring of PDMS (Sylgard 184, 10:1 ratio, cured 20 min at 120 °C) OD=25 mm, ID=15.5 mm in contact with the sensing side of the crystal and covered with 25 mm round No. 1 coverglass, nominal thickness 0.15 mm. The non-sensing side of the crystal remains in air and is isolated from the body of the centrifuge. The quartz crystals are always cleaned before use by immersion in fresh piranha solution (3:1 mixture of 97% H 2 SO 4 and 30% H 2 O 2 ) for 5 min and rinsing liberally with pure water. Free particles Free particles (Spherotech SVP-10-5, SVM-15-10, and SVP-200-4), of different diameters were prepared by diluting a solution of 30 μl particles in 300 μl H 2 O. A 125-μl aliquot of the 300 μl volume was then placed in the PDMS cell in contact with the sensing side of the crystal. The sensing area was calculated to be 1.195 cm 2 . The particles in solution experience a buoyant force, which reduces their apparent mass. The surface density N L was determined by counting the average number of particles per unit area with a microscope and was found to be within 20% of the value predicted by the volume concentration. Functionalization For experiments involving oligos, the crystals were first immersed in a 1-μM solution of thiolated oligos (5′-ThioMC6-TTT TTT TTT CAC TAA AGT TCT TAC CCA TCG CCC-3′) in a 1 M potassium phosphate buffer, 0.5 M KH 2 PO 4 , pH 3.8 for 1 h. Following, immersion in 1 mM 6-Mercapto-1-hexanol (MCH) was used to block residual reactive sites on the gold electrode. After rinsing, attachment to the prepared particles was done in STE buffer: 1 M NaCl with 10 mM Tris buffer, pH 7.4 and 1 mM EDTA. A complimentary strand (5′-biotin-CT CAC TAT AGG GCG ATG GGT AAG AAC TTT AGT-3′) was attached to the streptavidin-coated particles. The particles were first washed two times by aliquoting a 100-μl base solution of particles in 100 μl STE buffer, 5,000 r.p.m. for 3 min and decanting the supernatant. The particles were resuspended in 20 μl of STE buffer and 10 μg of oligos were added. The mixture was incubated for 15 min at room temperature under slow vortexing, then washed again and resuspended in 100 μl STE buffer. The oligo-attached particle suspension was allowed to attach to the gold surface for 15 min before spinning. Lambda DNAs were prepared by combining 50 μl of lambda DNA at 500 μg ml −1 , 5.5 μl of 10 × T4 ligase and 0.5 μl of diluted 10 μM thiolated linker oligonucleotide and heating to 70 °C for 5 min. The suspension was left to cool to room temperature as the litigation of the oligos to the DNA COS ends occured. Once the mixture was at room temperature, 15 μl 10 × ligase buffer, 127 μl H 2 O and 2 μl T4 DNA ligase were added to the annealed linker. The reaction was allowed to proceed at room temperature for 3 h. How to cite this article: Webster, A. et al. Probing biomechanical properties with a centrifugal force quartz crystal microbalance. Nat. Commun. 5:5284 doi: 10.1038/ncomms6284 (2014). Table 2 Results of the particle sizing method applied to particles with diameters and 25 μ m. Full size table